The four-transmembrane protein IP39 ofEuglenaforms strands by a trimeric unit repeat Euglenoid flagellates have striped surface structures comprising pellicles, which allow the cell shape to vary from rigid to flexible during the characteristic movement of the flagellates. In Euglena gracilis , the pellicular strip membranes are covered with paracrystalline arrays of a major integral membrane protein, IP39, a putative four-membrane-spanning protein with the conserved sequence motif of the PMP-22/EMP/MP20/Claudin superfamily. Here we report the three-dimensional structure of Euglena IP39 determined by electron crystallography. Two-dimensional crystals of IP39 appear to form a striated pattern of antiparallel double-rows in which trimeric IP39 units are longitudinally polymerised, resulting in continuously extending zigzag-shaped lines. Structural analysis revealed an asymmetric molecular arrangement in the trimer, and suggested that at least four different interactions between neighbouring protomers are involved. A combination of such multiple interactions would be important for linear strand formation of membrane proteins in a lipid bilayer. The PMP-22/EMP/MP20/Claudin superfamily comprises various membrane proteins with a four-transmembrane topology characterised by a large first extracellular loop containing a conserved W-LW-C-C motif and relatively short cytoplasmic loop and N-terminus [1] , [2] . Functional analyses suggested that these superfamily members are generally involved in cell-adhesion or transmembrane scaffolding in vertebrate epithelial and neuronal tissues [1] , [2] , [3] , [4] , [5] , [6] , and also in single-cell organisms [7] . Among these proteins, claudins have been well studied as major cell-adhesion molecules of tight junctions (TJs), which are typically localised at the uppermost portion of the lateral membrane in vertebrate epithelial and endothelial cells, and tightly connect adjacent cells to form paracellular barriers [8] , [9] . Freeze fracture electron microscopy revealed that claudin proteins are polymerised into a network of intramembrane particle strands at TJs [8] , [10] , [11] . Despite considerable interest in not only the adhesive properties but also in the processes of polymerisation into a one-dimensional array of claudin molecules, little information is available on the structure and oligomerisation states of any members of the superfamily, except for the bovine lens MP20 (ref. 12 ). Recently, the protozoan genes of the apparently 39-kDa integral membrane protein in Euglena gracilis were cloned [13] (GenBank Accession numbers: AB167379.1 and AB167380.1 ), and the protein was termed IP39 (refs 14 , 15 ). IP39 represents four predicted transmembrane domains and has a W-LW-C-C motif in the first extracellular loop, similar to the PMP-22/EMP/MP20/Claudin superfamily. IP39 is the most abundant membrane protein in the plasma membrane of Euglena gracilis [14] , [15] and has thus been studied as a major component of highly ordered intramembrane particles in the prominent striations observed in the freeze fracture replica [16] , [17] . Early studies reported that the striations or linear arrays of the IP39 molecules are not affected by isolation of the membrane fractions [16] or by trypsin digestion of the scaffolding proteins underneath the membrane [18] , implying that IP39 itself has a polymerising property to form linear and paracrystalline arrays. Here, we show the first three-dimensional (3D) structure of Euglena IP39 in a lipid bilayer, determined by electron crystallography of two-dimensional (2D) crystals. Our structure of the 2D crystal reveals a molecular strand comprising antiparallel double-rows, in which the trimeric units of the IP39 molecules are longitudinally polymerised. In the trimeric unit, one of the three protomers is rotated 180° in the opposite direction to the others, indicating a combination of multiple intermolecular interactions. Such an unexpected property of IP39 would be important for continuous linear polymerisation in Euglena membranes. These structural features also provide important implications for strand formation of the other four-transmembrane proteins of the PMP-22/EMP/MP20/Claudin superfamily. Crystallisation and 3D reconstruction of Euglena IP39 Euglena gracilis cells were grown in culture conditions and collected for large-scale purification. After alkaline treatment of the harvested cell membrane, IP39 was obtained as the major protein component, which was then solubilised with n-octyl-β- D -glucoside (OG) ( Supplementary Fig. S1a ). To remove the intrinsic lipids derived from the Euglena membrane, the solubilised supernatant was subjected to anion exchange chromatography and IP39 was further purified by NaCl gradient elution ( Fig. 1a , left). We verified that IP39 was phosphorylated in vivo , as previously described [19] , by immunoblotting with anti-phosphotyrosine antibody ( Fig. 1a , right). The purified IP39 showed monodispersity in size-exclusion chromatography ( Fig. 1b ) and was used for reconstitution into 2D crystals with 1,2-dioleoyl- sn -glycero-3-phosphocholine. Well-ordered crystalline vesicles with a width exceeding 1 μm were yielded by dialysis ( Fig. 1c ), and low-dose images were recorded from the frozen-hydrated samples by cryo-electron microscopy. The lattice constants of the 2D crystal were a =174.2 Å and b =59.3 Å, and the crystallographic symmetry was p2 ( Fig. 2a and Supplementary Table S1 ). A 3D electron microscopic density map (EM density map) of the IP39 crystal was reconstituted from images tilted up to 60° at around 10 Å resolution (see details in Methods and Supplementary Table S2 ) and showed that the molecular density layer was ~90 Å and contained one lipid bilayer in which the proteins were arranged ( Fig. 2b ). Each unit cell included 12 molecules, where 1 cluster of 6 molecules inserted into the lipid bilayer in the opposite direction to the other cluster of 6 molecules, due to the presence of pseudo-two-fold axes parallel to the b- axis in a unit cell ( Fig. 2a ). Each cluster extended repeatedly towards the b- axis, forming a double-row composed of two zigzag-shaped lines of molecules ( Fig. 3a ). We refer to one double-row as strand A, and the other as strand B. Strands A and B alternately aligned along the a- axis in a 2D crystal, exhibiting a novel type of molecular packing that appears like an array of polymers and not like an isotropic lattice. Although the two strands were not related by crystallographic symmetry, superposition of their respective density maps revealed quite similar structures with small differences in the regions protruding from the membranes ( Fig. 3c ). The differences could be due to mechanical contacts of the 2D crystals on the carbon support films during cryo-sample preparation by the carbon sandwich technique [20] , because the proteins were buried in large vesicular-form crystals ( Fig. 1c , inset) where the outer side of the vesicles attached to the upper and lower carbon film surfaces and the inner side of the vesicles faced the lumen and remained intact ( Supplementary Fig. S1b ). This is why p222 1 symmetry was not applied to the crystal, but both the A and B strands appeared to contain an equivalent arrangement of molecules. 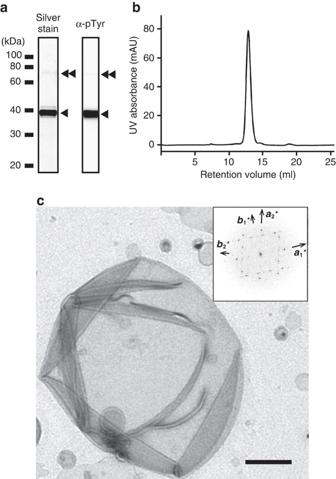Figure 1:EuglenaIP39 protein was purified and reconstituted into lipid for the 2D crystal. (a) Purified IP39 was separated by SDS–PAGE and analysed by silver staining (left) or western blotting probed with anti-phosphotyrosine antibody (right). The apparent molecular weight of the major band (single arrowhead) is ~39 kDa, consistent with previous studies. The faint bands at the higher molecular weight (double arrowhead) correspond to dimers. (b) Size-exclusion chromatography of the purified IP39 protein shows a monodisperse peak. (c) A negatively stained image of the vesicular 2D crystal of IP39, observed by conventional electron microscopy. The black bar represents 400 nm. (Inset) Fourier transform of the negatively stained 2D crystal. The two independent lattices (a1*b1* anda2*b2*) indicate overlapping of the upper and lower side crystals in the vesicle. Figure 1: Euglena IP39 protein was purified and reconstituted into lipid for the 2D crystal. ( a ) Purified IP39 was separated by SDS–PAGE and analysed by silver staining (left) or western blotting probed with anti-phosphotyrosine antibody (right). The apparent molecular weight of the major band (single arrowhead) is ~39 kDa, consistent with previous studies. The faint bands at the higher molecular weight (double arrowhead) correspond to dimers. ( b ) Size-exclusion chromatography of the purified IP39 protein shows a monodisperse peak. ( c ) A negatively stained image of the vesicular 2D crystal of IP39, observed by conventional electron microscopy. The black bar represents 400 nm. (Inset) Fourier transform of the negatively stained 2D crystal. The two independent lattices ( a 1 * b 1 * and a 2 * b 2 *) indicate overlapping of the upper and lower side crystals in the vesicle. 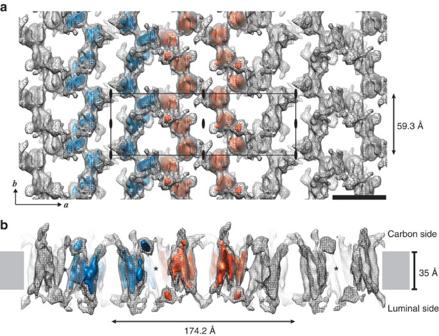Figure 2: 3D reconstructed structure of theEuglenaIP39 crystal. (a) 3D map of the IP39 crystal lattice viewed parallel to the two-fold axis from the luminal side of vesicular membrane. The grey mesh represents the EM density map contoured at 1.3σ. The internal molecular surfaces coloured blue and red represent two distinct pseudo-symmetric strands of the densities contoured at 3σ. The black box and closed ovals indicate a unit cell and two-fold symmetry axes, respectively. The right-angled arrows indicate the directions of thea- andb-axes. The black bar represents 50 Å. (b) Three-dimensional map viewed parallel to the membrane plane. Colour representations of the EM density map are the same as ina. The light grey bands represent the location of the lipid bilayer with a thickness of 35 Å. The asterisks indicate the pseudo two-fold axes along theb-axis. The numbers beside the double-headed arrows indicate the dimensions of a unit cell. Full size image Figure 2: 3D reconstructed structure of the Euglena IP39 crystal. ( a ) 3D map of the IP39 crystal lattice viewed parallel to the two-fold axis from the luminal side of vesicular membrane. The grey mesh represents the EM density map contoured at 1.3σ. The internal molecular surfaces coloured blue and red represent two distinct pseudo-symmetric strands of the densities contoured at 3σ. The black box and closed ovals indicate a unit cell and two-fold symmetry axes, respectively. The right-angled arrows indicate the directions of the a - and b -axes. The black bar represents 50 Å. ( b ) Three-dimensional map viewed parallel to the membrane plane. Colour representations of the EM density map are the same as in a . The light grey bands represent the location of the lipid bilayer with a thickness of 35 Å. The asterisks indicate the pseudo two-fold axes along the b -axis. The numbers beside the double-headed arrows indicate the dimensions of a unit cell. 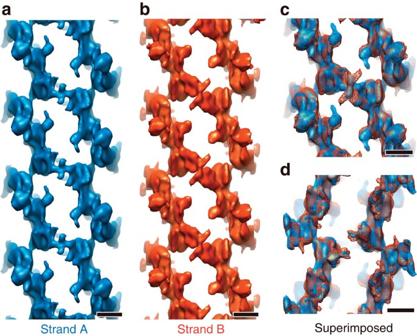Figure 3: Structural comparison of strands in the 2D crystal. (a,b) Molecular surfaces represent the isolated density maps of strand A viewed from the carbon side (a) and strand B viewed from the luminal side (b), contoured at 1.5σ. (c,d) EM density maps of strand A (blue surface) and strand B (red mesh) are superimposed and viewed perpendicular to the membrane plane from the luminal side (c) and the carbon side (d) for strand B. Colour codes are the same as inFig. 2. The black bars represent 20 Å. Full size image Figure 3: Structural comparison of strands in the 2D crystal. ( a , b ) Molecular surfaces represent the isolated density maps of strand A viewed from the carbon side ( a ) and strand B viewed from the luminal side ( b ), contoured at 1.5σ. ( c , d ) EM density maps of strand A (blue surface) and strand B (red mesh) are superimposed and viewed perpendicular to the membrane plane from the luminal side ( c ) and the carbon side ( d ) for strand B. Colour codes are the same as in Fig. 2 . The black bars represent 20 Å. Full size image Arrangement of IP39 molecules in a strand IP39 has four predicted transmembrane segments, and the size-exclusion chromatography profile and cross-linking experiments of the purified IP39 suggested that the protein was solubilised and stable as a monomer in the presence of OG ( Fig. 1b and Supplementary Fig. S1c ). In the 2D crystal, each strand contained apparently six molecules in a unit cell; within this unit, two clusters of three continuous molecules were related by two-fold symmetry ( Fig. 4a ). We refer to these molecules in the asymmetric unit as Mol1, Mol2 and Mol3 of strands A and B. To estimate the dimensions of the six molecules, each molecular density was isolated and the density, except for that in the putative transmembrane regions, was excised, and then the volume of the remaining density was measured because the regions outside the membrane layer varied between molecules. The mean volume of the density in the map at 0.8 σ was ~9500 Å 3 , equivalent to ~94% of the volume assumed from the 92 amino-acid residues in the predicted transmembrane regions (A-Mol1, 93%; A-Mol2, 99%; A-Mol3, 89%; B-Mol1, 97%; B-Mol2, 105%; B-Mol3, 82%; molecular mass was calculated by multiplying the volume by 0.81 Da Å −3 (ref. 21 )). This indicates that each molecule is likely a protomer of the IP39 protein and contains four transmembrane helices. Superposition of the isolated maps of the molecules in strand B (B-Mol1, Mol2 and Mol3; Fig. 4b ) revealed that all three molecules had the same features: one side was ‘pointed’ and the other side comprised ‘nock’ shapes perpendicular to the membrane plane ( Fig. 4c ). The three isolated densities were well fitted by correlation of the volume data values, and the larger protrusions in those ‘nock’ regions faced the same direction ( Fig. 4c ). The procedure for superposition of the molecules did not require an upside-down rotation to the membrane plane, but rather a rotation of ~180° of Mol3 around the axis perpendicular to the membrane plane for fitting. Also in strand A, all of the aligned molecules were inserted into the membrane in the same direction. Therefore, the structure of each strand might mimic the intrinsic molecular alignment of IP39 proteins in the native Euglena plasma membrane. 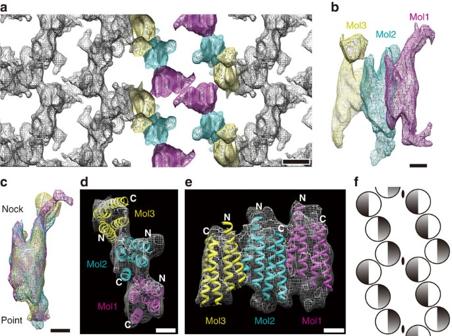Figure 4: Structural comparison of IP39 protomers. (a) EM density map containing approximately two unit cells is shown by mesh representation at 1.4σ, viewed from the luminal side. Unique molecular densities in strand B are coloured magenta (Mol1), cyan (Mol2) and yellow (Mol3). The molecules shown with the same colours are related by crystallographic symmetry. The black bar represents 20 Å. (b,c) Only the EM density of the three coloured molecules inaare shown by removing the other densities for clarity and viewed nearly parallel to the membrane plane (b). The three isolated molecules are superimposed (c) and the two sides of the densities are indicated as ’Nock‘ and ’Point‘. The black bars represent 10 Å. (d,e) Ribbon models of a four-helical bundle protein (PDB: 2UUI) are fitted to the EM density map (light grey mesh contoured at 1.3σ, putative transmembrane region only) of the three molecules in strand B. The fitted model helices are represented by magenta, cyan and yellow ribbons superimposed on Mol1, 2 and 3, respectively, viewed perpendicular (d, from the same direction witha) and parallel (e, the upper side is the ’Nock‘ side) to the membrane plane. The white bars represent 10 Å. (f) A schematic diagram representing the arrangement, directions and spacing of the IP39 protomers in a single strand viewed perpendicular to the membrane plane by the black and white circles. The black semicircular side indicates the large protruding side in the cytosolic region of the IP39 proteins. Figure 4: Structural comparison of IP39 protomers. ( a ) EM density map containing approximately two unit cells is shown by mesh representation at 1.4σ, viewed from the luminal side. Unique molecular densities in strand B are coloured magenta (Mol1), cyan (Mol2) and yellow (Mol3). The molecules shown with the same colours are related by crystallographic symmetry. The black bar represents 20 Å. ( b , c ) Only the EM density of the three coloured molecules in a are shown by removing the other densities for clarity and viewed nearly parallel to the membrane plane ( b ). The three isolated molecules are superimposed ( c ) and the two sides of the densities are indicated as ’Nock‘ and ’Point‘. The black bars represent 10 Å. ( d , e ) Ribbon models of a four-helical bundle protein (PDB: 2UUI) are fitted to the EM density map (light grey mesh contoured at 1.3σ, putative transmembrane region only) of the three molecules in strand B. The fitted model helices are represented by magenta, cyan and yellow ribbons superimposed on Mol1, 2 and 3, respectively, viewed perpendicular ( d , from the same direction with a ) and parallel ( e , the upper side is the ’Nock‘ side) to the membrane plane. The white bars represent 10 Å. ( f ) A schematic diagram representing the arrangement, directions and spacing of the IP39 protomers in a single strand viewed perpendicular to the membrane plane by the black and white circles. The black semicircular side indicates the large protruding side in the cytosolic region of the IP39 proteins. Full size image To examine the arrangement of each molecule in the trimeric unit, we attempted to find a well-fitted template structure to our EM map from the known structures of the four-helical bundle of the membrane proteins selected by manual inspection from the database SCOP [22] and membrane proteins of a known 3D structure ( http://blanco.biomol.uci.edu/mpstruc/listAll/list ) ( Fig. 4d ). Twelve models, including connexin26 and the K subunit of V-type ATPase, were selected to dock into the EM map using the Situs program [23] . The model best fitted to the density of the IP39 protomer (the cross-correlation function: 0.816 to B-Mol1, 0.857 to B-Mol2 and 0.838 to B-Mol3) was the structure of leukotriene C4 synthase (Protein Data Bank ID: 2UUI), which had a MAPEG domain-like fold. Although the TM1 of Mol1 faced the TM4 of Mol2, the TM1 of Mol2 was adjacent to the TM1 of Mol3. This was the result of a 180° rotation to fit the model to the density of Mol3 ( Fig. 4d ). Such different orientations between each molecule in the unit led to particularly unique contacts between adjacent units ( Fig. 4f ). Each optimal position in the unit was further refined by collage in Situs (overall cross-correlation function: 0.833). These findings also indicate that the asymmetric trimer is the minimal unit of the strands in the IP39 crystal, even though the IP39 molecules exist as monomers in the OG-solubilising state before crystallisation. This was further supported by western blotting results of the Euglena membrane fraction before solubilisation, which showed prominent bands corresponding to the dimer and trimer of IP39 as well as the monomer ( Supplementary Fig. S1a ). Determination of the intracellular and extracellular sides In the 2D crystal, membrane protein molecules are buried in a lipid bilayer, exposing the intracellular and extracellular regions to an aqueous environment. The IP39 protomers in the 2D crystal had prominent protrusions extended from the ‘nock’ regions ( Fig. 4b ). The bridge-like protrusions of the two Mol1 protomers connected the two zigzag-shaped lines of the molecules in a strand ( Fig. 3a–c and Fig. 4a ). In the EM map of our crystal structure, however, we were unable to determine whether the protrusions belonged to the intracellular side or extracellular side because the regions of the intracellular side with N- and C-termini and those of the extracellular side with the long loop could not be clearly distinguished. To determine the sidedness in the map, we added the Fab fragments of anti-phosphotyrosine antibodies against the IP39 crystals for intracellular labelling and obtained images of the Fab-bound crystals using cryo-electron microscopy. The ability of the antibodies to attach to the crystals was confirmed by gold-conjugated secondary antibody labelling and negative staining ( Supplementary Fig. S2a ). Compared with the projection map merged from non-tilted images of Fab-free IP39 crystals, the densities between the two lines in either strand A or B were reduced in the map of Fab-bound IP39 crystals ( Fig. 5a ; red arrows). Furthermore, 3D reconstruction from a series of images tilted to 45° was compared with 3D reconstruction from images of Fab-free IP39 crystals similarly tilted to 45°, showing the disappearance of the bridge-like densities between only the A-Mol1 protomers, probably due to disordering by attachment of the Fab fragments ( Fig. 5c ; red arrows). The densities of the same protrusions on the opposite side of strand B were not altered ( Fig. 5c ; black arrows), because the Fab fragments could not permeate the membrane layers or access the epitope regions that were facing the lumen of the vesicular crystal ( Supplementary Fig. S2c ). As phosphorylation is a modification specific to cytosolic amino-acid residues, bridge-like regions showing the difference by the Fab addition should belong to the intracellular side. Though each protomer should have a phosphorylated cytosolic region, there was no apparent difference in the Mol2 and Mol3 protomers other than the densities extended from Mol1 protomers. This implies that the regions including the phosphorylated tyrosine residues were flexible and thus likely to be also disordered in the original crystal structure. The secondary structure of the IP39 amino-acid sequences potentially indicates that there are cytosolic tyrosine residues only at the C-terminal tail ( Supplementary Fig. S3 ). Therefore, in the 2D crystal, some of the tyrosine residues are phosphorylated and may be included in the flexible, unstructured regions of the C-terminal protrusions or the bridge-like regions between the Mol1 protomers. 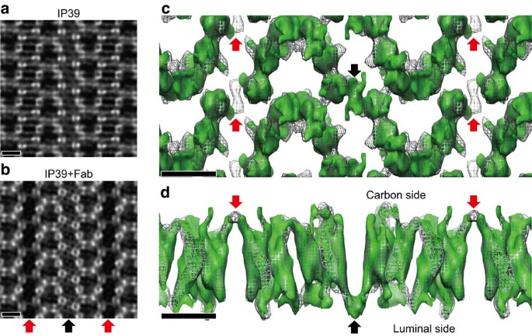Figure 5: Anti-phosphotyrosine Fab antibody distinguishes the intracellular side of the IP39 structures. (a,b) Projection maps merged from the non-tilted images of IP39 crystals (a) and IP39 crystals with Fab fragments of anti-phosphotyrosine antibody (b). Red arrows indicate the prominent disappearance of the lines of the projection densities with the addition of Fab. The black bars represent 40 Å. (c,d) Three-dimensional maps reconstituted from 0–45° images of IP39 crystals (grey mesh) and IP39 crystals with Fab fragments of anti-phosphotyrosine antibody (green surface) are superimposed. The resolution limits of the two maps are cutoff at 10 Å. The EM maps are viewed perpendicular (c, from the luminal side) and parallel (d) to the membrane plane. Red and black arrows indicate the regions of the bridge-like protrusion in strands A and B, respectively. The black bars represent 40 Å. Figure 5: Anti-phosphotyrosine Fab antibody distinguishes the intracellular side of the IP39 structures. ( a , b ) Projection maps merged from the non-tilted images of IP39 crystals ( a ) and IP39 crystals with Fab fragments of anti-phosphotyrosine antibody ( b ). Red arrows indicate the prominent disappearance of the lines of the projection densities with the addition of Fab. The black bars represent 40 Å. ( c , d ) Three-dimensional maps reconstituted from 0–45° images of IP39 crystals (grey mesh) and IP39 crystals with Fab fragments of anti-phosphotyrosine antibody (green surface) are superimposed. The resolution limits of the two maps are cutoff at 10 Å. The EM maps are viewed perpendicular ( c , from the luminal side) and parallel ( d ) to the membrane plane. Red and black arrows indicate the regions of the bridge-like protrusion in strands A and B, respectively. The black bars represent 40 Å. Full size image Combination of multiple intermolecular interactions in a strand Based on the structural features of the 2D crystal of the IP39 molecules, as well as the structural analysis of the immuno-labelled 2D crystals, electron crystallography revealed that multiple interactions occur to form the straight strand of Euglena IP39. In the single strand, the four distinct interaction patterns between IP39 protomers can be classified as Mol1–Mol2, Mol2–Mol3, Mol3–Mol1 and Mol1–Mol1 interactions ( Fig. 6 ). First, the interactions at the transmembrane regions are crucial ( Fig. 6b–d ), and a pair of homogeneous IP39 protomers can form intermolecular interactions at different sets of transmembrane sites. Second, in the Mol2–Mol3 interaction, protrusion of the Mol3 cytosolic region overlays a non-protruding part of the cytosolic region of Mol2 ( Figs 4a,b and 6c ). This implies the involvement of the cytosolic region in the strand formation in the interaction of this specific pair. Finally, the Mol1–Mol1 interaction links the two antiparallel lines of the molecules at the cytosolic protrusions, referred to as a ‘bridge’ whose density was clearly observed at the intracellular side between Mol1–Mol1 ( Fig. 6e ). The regular order of the combination of these interactions provides the basis for the strand formation by polymerisation of the IP39 molecules. 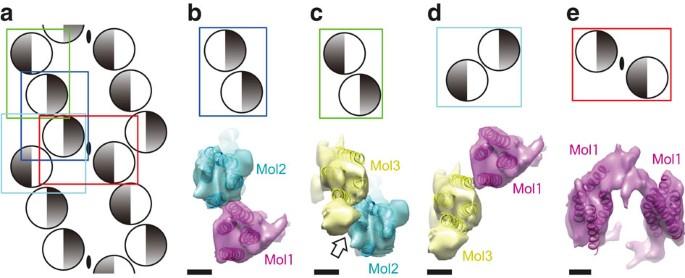Figure 6: Combination of four different interaction modes forms a linear strand. (a) A schematic diagram showing the arrangement of the IP39 protomers as shown inFig. 4f. The four coloured rectangles distinguish the different pairs of interacting molecules. (b–e) The respective pairs of molecules shown inaare extracted (upper panels) and the corresponding EM density maps are represented by transparent surfaces with the fitted model helices superimposed (lower panels). The maps of Mol1-Mol2 (b), Mol2-Mol3 (c) and Mol3-Mol1 (d) are viewed perpendicular to the membrane planes from their intracellular sides, and the map of Mol1-Mol1 (e) is viewed slightly diagonally from the intracellular side. The black open arrow indicates the overlaid area of the Mol3 protrusion on the cytosolic region of Mol2. The surface colour codes are the same as inFig. 4a. The black bars represent 10 Å. Figure 6: Combination of four different interaction modes forms a linear strand. ( a ) A schematic diagram showing the arrangement of the IP39 protomers as shown in Fig. 4f . The four coloured rectangles distinguish the different pairs of interacting molecules. ( b – e ) The respective pairs of molecules shown in a are extracted (upper panels) and the corresponding EM density maps are represented by transparent surfaces with the fitted model helices superimposed (lower panels). The maps of Mol1-Mol2 ( b ), Mol2-Mol3 ( c ) and Mol3-Mol1 ( d ) are viewed perpendicular to the membrane planes from their intracellular sides, and the map of Mol1-Mol1 ( e ) is viewed slightly diagonally from the intracellular side. The black open arrow indicates the overlaid area of the Mol3 protrusion on the cytosolic region of Mol2. The surface colour codes are the same as in Fig. 4a . The black bars represent 10 Å. Full size image Our crystal structure of the purified IP39 protein revealed that IP39 polymerised to form a linear strand with two anti-parallel lines of molecules, a so-called molecular strand. Stabilisation of the linearity by the antiparallel arrangement of the two lines is more reminiscent of a DNA double helix than an actin filament [24] . Membrane proteins, however, are unable to form a helical arrangement such as those formed by filaments, owing to the spatial restriction in the 2D plane. The simplest way to form a strand in the membrane plane is to align molecules to be straight and unidirectional in a single file, but because the long row of polymerised molecules becomes flexible and will lean away from the centreline, such a simple alignment method would result in a circular oligomerisation, such as the rotor ring (‘K-ring’) of the V-type ATPase from Enterococcus hirae [25] where the 10 subunits of the four-transmembrane polypeptides form a circular rotor domain. In the case of the IP39 strand, alternatively, the key solution is that intermittently one of the three molecules, in this case Mol3, rotates in the opposite direction and resets the distortion of the line ( Fig. 4d ). Although the precise interaction sites or residues involved in the polymerisation could not be determined with our map of the crystal, the close fit of the model helices with the EM map implied that the interactions between transmembrane regions are crucial for this unique arrangement ( Fig. 4d,e and 6b–d ), and it should be noted that the pair of homogenous IP39 protomers can form intermolecular interactions at different sets of transmembrane sites. Furthermore, in the Mol2–Mol3 interaction, the protrusion of the Mol3 cytosolic region extends over the non-protruding side of the Mol2 cytosolic region ( Fig. 6c ), which implies the involvement of the cytosolic region in the strand formation by a specific interaction with the soluble parts. The regular order of the combination of such multiple interactions would be the basis for the linear and continuous strand formation by polymerisation of the IP39 molecules. With such a continuous strand, a cell membrane could be separated into different areas and also cells could form a continuous tightly sealed junction, such as the TJs formed by claudin [8] . In the native Euglena gracilis membrane, these strands are arranged sideways and form a lattice, which may be stabilised by more interactions between the neighbouring strands, but such interactions could not be explained in the 2D crystal because of the upside-down abreast arrangement of the strands ( Fig. 2b ). This upside-down arrangement in the 2D crystal, however, suggests that the inter-strand interactions might be relatively weak, allowing the Euglena to have a somewhat flexible membrane. The euglenoid movement is a characteristic motility for the euglenoid flagellates, involving changing the shape of their bodies, which enables the single-cell organisms to swim without waving their flagella [26] , [27] . The pellicular structures are commonly observed on the surface of the organisms and should be responsible for the movement [28] , [29] . During the movement, the adjacent pellicular strips slide past each other, maintaining the width and length of the strips [27] , [30] . In Euglena gracilis , the IP39 proteins are the highly ordered intramembrane particles restricted in the ridge regions of the pellicular membranes [14] , [16] and bound to submembrane cytoskeletons [18] , [31] , and thus may have a stabilizing role for maintaining the strength of the membrane to couple motive forces of the movement with the pellicular sliding. The EM map of our crystal structure revealed a unique arrangement of the IP39 molecules for strand formation in the membrane, implying a functional role in both the rigidity and flexibility of the pellicular strips in Euglena gracilis . In contrast to the concave groove regions, which are devoid of intramembrane particles [16] , [32] , IP39 polymers cover the entire ridge regions and should not only maintain the strip of membrane against a rapid change in its overall shape during euglenoid movement, but also have an elastic property, similar to a spring, to form the slightly curved shape of the pellicular ridge, probably due to the zigzag arrangement of the molecules. Slight sliding at the interface of neighbouring strands and compression of parallel pairs of the zigzag rows could account for a certain degree of flexibility of the strand arrangement when required for flagellate movement. IP39 is a tetra-spanning membrane protein and has a similar overall topology with the PMP-22/EMP/MP20/Claudin superfamily and shares the well-conserved sequence motif in the first extracellular loop ( Supplementary Figs S3, S4 ), although the biological functions of this newly identified member of the superfamily must be examined by further biochemical and cell biological studies. Each member in this superfamily has distinct functions, but is considered to share some kind of adhesive role in the membrane [1] . MP20, which is the second most prevalent membrane protein of the lens fibre cells, was suggested to form the rectangular octamer comprising two asymmetric units in the 2D crystal lattice, revealed in the projection map by negative stain EM [12] . It is likely that MP20 forms an isotropic lattice, because MP20 has a potential role in junctional organisation [33] and is dispersedly distributed in the lens fibre cell membrane [34] . In contrast, IP39 forms an anisotropic lattice in the 2D crystal, which may be due to its intrinsic properties that it forms linear strands, implying that the TJ strands that mainly comprise claudin proteins are similar in molecular arrangement [1] , [8] . Further studies are needed to elucidate how multiple interactions occur in the four-helix proteins and how the regular order of the multiple interactions proceeds. This study revealed for the first-time the 3D structure of a membrane protein to form a continuous strand that could be common in the PMP-22/EMP/MP20/Claudin superfamily. Purification of Euglena IP39 Euglena gracilis was grown in Koren–Hutner medium [35] , which was slightly modified (major constituents (g l −1 ): L -arginine HCl 0.5; L -aspartic acid 0.3; glucose 12.0; L -glutamic acid 4.0; glycine 0.3; L -histidine HCl·H 2 O 0.05; DL-malic acid 6.5; Na 3 citrate·H 2 O 0.58; Na 2 succinate 0.1; (NH 4 ) 2 SO 4 0.5; NH 4 HCO 3 0.25; KH 2 PO 4 0.25; MgCO 3 0.6; CaCO 3 0.12. minor constituents (mg l −1 ): EDTA-Na 2 50.0; FeSO 4 (NH 4 ) 2 SO 4 ·6H 2 O 50.0; MnSO 4 ·H 2 O 18.0; ZnSO 4 ·7H 2 O 25.0; (NH 4 ) 6 Mo 7 O 24 ·4H 2 O 4.0; CuSO 4 1.2; NH 4 VO 3 0.5; CoSO 4 ·7H 2 O 0.5; H 3 BO 3 0.6; NiSO 4 ·6H 2 O 0.5; thiamine-HCl 2.5; cyanocobalamin 0.005) at 60 r.p.m. in an Erlenmeyer flask at 27 °C. Harvested cells were washed and pelleted in 100 mM Tris (pH 7.5), 10 mM EGTA. Cells were disrupted by sonication in 1 mM Tris (pH 7.5), 0.1 mM EGTA, 10 μM leupeptin and 0.5 mM phenylmethylsulfonyl fluoride, and crude membrane was collected by centrifugation at 2,000 g for 20 min. Crude membrane was homogenised with 10 mM NaOH and a membrane fraction containing IP39 was obtained by ultracentrifugation at 131,000 g for 20 min. Alkaline-washed membranes were neutralised in 10 mM Tris (pH 7.5) and solubilised with 10% (w/v) OG (Dojindo) for 30 min at 4 °C. Insoluble materials were removed by ultracentrifugation at 100,000 g for 10 min and the OG-solubilised fraction was injected into a HiTrap Q HP anion exchange column (GE Healthcare) pre-equilibrated with 2% OG and 10 mM Tris (pH 7.0). IP39 was eluted in 2% OG, 10 mM Tris (pH 7.0) and a 20–250 mM NaCl gradient. At the anion-exchange chromatography step during purification, IP39 proteins were separated as multiple peaks depending on their phosphorylation status, consistent with the results of 2D-PAGE in a previous report [19] . The fractions containing phosphorylated IP39 were collected and used for 2D crystallisation. Monodispersity of the purified sample was checked by size-exclusion chromatography using a Superdex 200 10/300 column (GE healthcare) with 2% OG and 10 mM Tris (pH 7.0). Purified protein was analysed by SDS–PAGE and N-terminal amino-acid sequencing (APRO Science), and the N-terminal sequence was determined as Ala-Gly-Gly-Pro-Val, confirming that the obtained protein was IP39, with an N-terminal methionine excised ( Supplementary Fig. S3 ). 2D crystallisation Purified IP39 was adjusted to a concentration of 0.35 mg ml −1 and mixed with 1,2-dioleoyl-sn-glycero-3-phosphocholine (Avanti Polar Lipids) at a lipid-to-protein ratio (w/w) of 0.45 to 0.55. The mixture was placed in 15-μl microdialysis button (Hampton Research) using a dialysis membrane with a molecular weight cutoff of 15 kDa (SPECTRA/Por no. 7, SPECTRUM) and dialysed for 3 days in 10 mM Hepes (pH 7.0), 150 mM NaCl, 1 mM MgCl 2 and 30% (v/v) glycerol. During dialysis, the temperature was kept at 20 °C on the first day, 37 °C on the second day and 20 °C on the third day. Electron microscopy and image analysis Samples were negatively stained with 2% (w/v) uranyl acetate for conventional electron microscopy. For cryo-electron microscopy, specimens were prepared using the carbon sandwich method [20] . Briefly, a 2D crystal sample was mixed with buffer containing 10 mM Hepes (pH7.0), 1 mM MgCl 2 and 7% (w/v) trehalose on a molybdenum grid with a first carbon film. The solution was then removed, and the grid was washed with the buffer described above to remove residual salt and glycerol before covering with a second carbon film. Excess buffer was blotted from the side of the grid using filter paper and the grid was plunged into liquid nitrogen. All steps were performed at 4 °C. Images were recorded using a JEM-3000SFF electron microscope (JEOL) equipped with a field emission gun and a super-fluid helium stage [36] at an acceleration voltage of 300 kV. Low-dose images of the crystals at tilt angles of 0–60° were recorded on Kodak SO-163 film (Carestream Health) at a nominal magnification of × 40,000. The quality of the images was assessed by optical diffraction, and selected images were digitized with a SCAI scanner (Zeiss) using a step size of 7 μm. The digitized images, typically 5,000 × 5,000 pixels, were processed with the MRC image processing programs [37] . The crystals were computationally unbent and corrected for the contrast transfer function [38] . The initial contrast transfer function parameters for each image were determined by square frequency filtering [39] combined with periodogram averaging [40] . The data from 310 images were combined using LATLINE [41] and used to calculate a density map at 7 Å resolution ( Supplementary Table S2 ). It is notable, however, that each 2D crystal of IP39 gave anisotropic diffraction in the plane of the membrane ( Supplementary Fig. S5a,b ). In X-ray crystallography, diffraction anisotropy was sometimes observed and processed with an ellipsoidal truncation [42] . To determine the effective resolution of our map, we plotted the averaged F/sigma of reflections from the merged data for the unit cell axis of the 2D crystal ( Supplementary Fig. S6 ). The plot showed that the averaged F/sigma along the b * direction decreased more rapidly than that along the a * direction. Taking into consideration the plot and the effect of map calculations with limited indices, we estimated the maximum resolutions at 8.3, 11.9 and 8.3 Å along the a *-, b *- and c *-axis, respectively. Owing to anisotropy in the plane of the membrane, the calculated EM density map had elongated features along the b- axis ( Supplementary Fig. S7 ). As such features were more enhanced by B-factor sharpening [43] , we used the original EM map. Initial symmetry assignments were performed with ALLSPACE [44] ( Supplementary Table S1 ). The symmetry candidates were p1 , p2 , p12 1 a or p222 1 b . Judging from the IQ-plot calculated from the non-tilted images, symmetry 2 1 was often destroyed because of the mechanical contact of the 2D crystals with the carbon support films during cryo-sample preparation (see Supplementary Fig. S5a and the legend). The correct symmetry was only confirmed by building the 3D reconstruction without imposing symmetry. The IQ-weighted phase residuals of the reconstituted structure calculated at 10 Å resolution were 28.9°, 32.4° and 51.2° in the p1 , p2, and p222 1 symmetries, respectively. Therefore, the p2 symmetry was confirmed. All figures of the 3D EM density maps were drawn by UCSF Chimera [45] . Model fitting The candidate transmembrane model of IP39 was selected from the known structures of four-helical bundles of membrane proteins from the database SCOP [22] and membrane proteins with a known 3D structure (http://blanco.biomol.uci.edu/mpstruc/listAll/list). After selection by manual inspection, 12 models were selected: F 1 F O ATP synthase subunit A (PDB: 1C17), neurotransmitter-gated ion-channel transmembrane pore (PDB: 1OED), heme-binding four-helical bundle (PDB: 1PPJ, 1KQF, 1Q16, 2BS2, 1NEK), MAPEG domain-like (PDB: 2Q7R, 2H8A, 2UUI), connexin26 (PDB: 2ZW3) and V-ATPase K-ring (PDB: 2BL2). The transmembrane regions of these models were used to dock into the EM map by Situs [23] . The model best fitted to the density corresponding to the IP39 monomer in EM map was the structure of leukotriene C4 synthase (PDB: 2UUI). Further positional refinements in the unit were then performed by collage in Situs. Fab preparation and labelling Anti-phosphotyrosine antibody (PY20) was purchased from Millipore. Fab fragments of PY20 were generated and purified using Fab Preparation Kit (Pierce) according to the manufacturer’s protocol. Purified Fab fragments were added to IP39 crystals at a final concentration of 0.35 mg ml −1 and incubated at 4 °C overnight. Fab-labelled crystals were frozen and preserved in liquid nitrogen after carbon sandwich preparation and used for cryo-electron microscopy. Low-dose images of the crystals at tilt angles of 0–45° were recorded and analysed in the same way as those of the crystals without Fab ( Supplementary Table S3 ). Accession codes: Coordinates and EM density maps for IP39 and Fab-bound IP39 have been deposited in the EMDataBank under accession codes EMD-2314 and EMD-2315. How to cite this article: Suzuki, H. et al . The four-transmembrane protein IP39 of Euglena forms strands by a trimeric unit repeat. Nat. Commun. 4:1766 doi: 10.1038/ncomms2731 (2013).